Stereoselectivity and electrostatics in charge-transfer Mn- and Cs-TCNQ4networks on Ag(100) Controlling supramolecular self-assembly is a fundamental step towards molecular nanofabrication, which involves a formidable reverse engineering problem. It is known that a variety of structures are efficiently obtained by assembling appropriate organic molecules and transition metal atoms on well-defined substrates. Here we show that alkali atoms bring in new functionalities compared with transition metal atoms because of the interplay of local chemical bonding and long-range forces. Using atomic-resolution microscopy and theoretical modelling, we investigate the assembly of alkali (Cs) and transition metals (Mn) co-adsorbed with 7,7,8,8-tetracyanoquinodimethane (TCNQ) molecules, forming chiral superstructures on Ag(100). Whereas Mn-TCNQ 4 domains are achiral, Cs-TCNQ 4 forms chiral islands. The specific behaviour is traced back to the different nature of the Cs- and Mn-TCNQ bonding, opening a novel route for the chiral design of supramolecular architectures. Moreover, alkali atoms provide a means to modify the adlayer electrostatic properties, which is important for the design of metal–organic interfaces. Self-assembly provides a very promising bottom–up fabrication strategy that has been employed in many different fields like organic electronics, crystal engineering and design of hybrid nanocomposite materials [1] , [2] , [3] , [4] , [5] . This idea takes inspiration from nature itself: perhaps the most comprehensive and impressive display of the self-assembly potential for both reproducibility and scalability is found in biological systems, where long-range van der Waals and electrostatic interactions typically drive very complex stereoselective assembly processes. These may, for example, involve proteins or nucleic acid strands that are chiral assemblies of smaller units such as amino acids and nitrogenous bases. Stereoselective assembly in the presence of long-range interactions also occurs in much simpler molecular systems adsorbed on a substrate [6] , [7] , [8] , [9] , where it is readily accessible to direct experimental observation [10] , [11] . For instance, the crystallization of a mixture of chiral molecules in bulk compounds, or on a surface, typically results either in the formation of racemates, that is, crystals having a unit cell containing two different enantiomers, or in the separation of enantiomers forming crystals of a single-handedness, known as racemic conglomerates [12] . Clearly, if appropriately rationalized, this vast repertoire of assembly behaviours could be used to build and tune the properties of metal–organic interfaces. However, the specific behaviour of a particular chiral molecule is generally difficult to predict [13] and must be experimentally determined. Scanning tunnelling microscopy (STM) imaging at submolecular resolution has offered a great deal of information on the local structure, chiral organization, separation and recognition of both intrinsically chiral and prochiral molecules on surfaces [14] , [15] , [16] , [17] , [18] , [19] . Interestingly, experiments have revealed that the enantiomer units may be intermediate chiral assemblies of smaller achiral molecules [20] , and may even form on mirror symmetric (non-chiral) substrates such as high-symmetry noble metal surfaces [21] . This is the special case addressed in the present work, in which racemate formation or chirality segregation emerge purely as a result of symmetry-breaking mechanisms determined by energy considerations, depending on the specific steric constraints associated with the inter-molecular linkage network in the presence of different bridging metal atom species. In many previous studies, the use of transition metal bridging atoms linking organic molecules on mirror symmetric substrates has emerged as a tool to achieve control of the assembled structures [22] , [23] , [24] . The use of alkali metals in the same context has been much less explored [25] , [26] , although their low ionization energy may induce charging processes and lead to a potentially interesting interplay between local linkage and long-range electrostatic effects. The latter are very important because, for example, the formation of surface electric dipoles would allow some control of the interface level alignment, one of the main issues in organic electronics [27] . However, a generally accepted picture of interfacial level alignment is still missing: while the surface dipole formation as a function of the substrate work function and adsorbed organic molecule species has been extensively explored, no reliable recipe has been proposed to predict the dipole formation and the associated electric potential offset that controls the surface work function variations. As a consequence, device design is still often a trial-and-error process [28] . In this context, the investigation of the assembly behaviour of charged organic molecules and different metal linkage atoms on metal substrates can help in clarifying and tuning some functional properties of metal-organic interfaces. Here we investigate the chiral and electrostatic properties of metal–organic superstructures obtained from achiral tetracyanoquinodimethane (TCNQ) molecules co-deposited with Cs and Mn metal atoms on the Ag(100) surface, by means of STM and density functional theory (DFT) calculations. We find that both Mn and Cs adatoms yield the formation of intermediate chiral metal–TCNQ 4 windmill complexes. However, while Mn–TCNQ 4 assemble into achiral domains ( Fig. 1a,b ), Cs–TCNQ 4 induce strictly chiral domains that are also much more extended ( Fig. 1c–e ) and allow a regular lattice of empty holes that could serve as contact sites with the substrate across the organic layer. Our results show that these differences are a consequence of the dissimilar nature of the Cs– and Mn–ligand bonding. From the chemical point of view, choosing Cs (an alkali atom, forming ionic complexes) over Mn (a transition metal atom, forming directional square coordination complexes) induces significant differences in the stiffness of the resulting metal–TCNQ 4 complex. This local chemical bonding behaviour translates into distinctly different chiral adlayer organizations. In terms of electrostatics, the choice of Cs, with its strong donor character, promotes the formation of a stable organic salt layer resulting in a local electric dipole profile very different from the one found for Mn–TCNQ 4 . This is possible because the Cs cation is not bound to the horizontal plane of its four ligands, a fact that gives further reason for the enhanced stability of the Cs-bound monolayer. 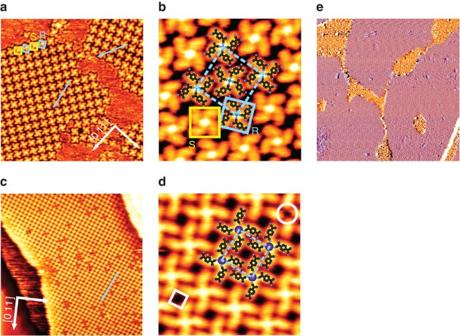Figure 1: STM data of self-assembled metal–TCNQ complexes on Ag(100). (a,b) Mn–TCNQ4achiral superstructure: (a) 48×48 nm2size STM image showing two non-equivalent achiral domains, mirror symmetric with respect to the [011] substrate direction. Alternating yellow and blue squares symbolize clockwiseR- and anti-clockwiseS-enantiomers, respectively. (b) Detailed image (8×8 nm2) of the arrangement of the complexes. The superstructure square unit cell size is 27.4 Å, whereas the Mn–Mn nearest-neighbour distance is 19.4 Å. (c,d) Cs–TCNQ4chiral superstructure: (c) large-scale image showing a single domain ofS-enantiomers (image size 73×73 nm2). The blue (white) arrow indicates the superstructure domain orientation (substrate [011] orientation). CoexistingR-domains are observed elsewhere on the surface. (d) Detailed image (8×8 nm2) of the domain structure. The dashed blue square marks the superstructure unit cell, corresponding to a Cs–Cs distance of 19.4 Å. The white circle indicates a Cs vacancy, and the white square marks one of the regularly spaced square-shaped holes in the superstructure. (e) Derivative of STM image showing large domains of chiral Cs–TCNQ4networks (highlighted in pink, image size 330×330 nm2). Figure 1: STM data of self-assembled metal–TCNQ complexes on Ag(100). ( a , b ) Mn–TCNQ 4 achiral superstructure: ( a ) 48×48 nm 2 size STM image showing two non-equivalent achiral domains, mirror symmetric with respect to the [011] substrate direction. Alternating yellow and blue squares symbolize clockwise R - and anti-clockwise S -enantiomers, respectively. ( b ) Detailed image (8×8 nm 2 ) of the arrangement of the complexes. The superstructure square unit cell size is 27.4 Å, whereas the Mn–Mn nearest-neighbour distance is 19.4 Å. ( c , d ) Cs–TCNQ 4 chiral superstructure: ( c ) large-scale image showing a single domain of S -enantiomers (image size 73×73 nm 2 ). The blue (white) arrow indicates the superstructure domain orientation (substrate [011] orientation). Coexisting R -domains are observed elsewhere on the surface. ( d ) Detailed image (8×8 nm 2 ) of the domain structure. The dashed blue square marks the superstructure unit cell, corresponding to a Cs–Cs distance of 19.4 Å. The white circle indicates a Cs vacancy, and the white square marks one of the regularly spaced square-shaped holes in the superstructure. ( e ) Derivative of STM image showing large domains of chiral Cs–TCNQ 4 networks (highlighted in pink, image size 330×330 nm 2 ). Full size image Formation of metal-TCNQ 4 complexes on Ag(100) The STM images of the metal–organic structures after deposition of Mn and Cs on the TCNQ adlayer show domains of closely packed mononuclear windmill-shaped units as shown in Fig. 1a–d , respectively. The complexes consist of a central protrusion representing the metal atom, surrounded by four TCNQ molecules aligned perpendicularly to each other. Although the individual Cs and Mn complexes appear similar in structure, their organization in extended superstructures strongly depends on the metal atom at their centre. In the achiral Mn–TCNQ 4 network two non-equivalent domain orientations can be identified ( Fig. 1a ). The domains consist of alternating R and S enantiomers ( Fig. 1b ), and are mirror-symmetric with respect to the [011] substrate direction (oriented at ~±(19°±2°), where the orientation is defined connecting next-nearest neighbour Mn atoms). The size of the unit cell is (28.1±1) Å ~9.5 a 0 , corresponding approximately to a (9, 3/−3, 9) commensurate superstructure ( a 0 =2.89 Å is the Ag(100) nearest-neighbour distance). TCNQ molecules within R / S Mn–enantiomers have their long axes oriented +19°/−19° (±3°) with respect to [011] (ref. 24 ). In contrast, Cs–TCNQ 4 forms large domains (>200 nm) and both individual chiral complexes and domains are mirror symmetric with respect to [011] ( Fig. 1c–e ). The square unit cell has a lattice constant of (19.4±1) Å ~6.7a 0 , indicating a commensurate (6, 3/−3, 6) superstructure. The R / S domain orientation forms an angle of +26.7°/−26.7° (±2°) with respect to the [011] principal surface directions. Figure 1c shows an S -domain. The coexisting R -domains were observed elsewhere on the surface. As in Mn–TCNQ 4 domains, the TCNQ molecules within a R / S unit are adsorbed with their long axis forming a +19°/−19° (±3°) angle with [011]. Thus, the two equivalent supramolecular adsorption configurations lead to opposite enantiomers on binding to the metal atoms. Unlike in the Mn–TCNQ 4 case, the compact arrangement leaves regularly spaced holes with an apparent size of about 6.3×6.3 Å 2 in the Cs co-adsorbed adlayer ( Fig. 1d ). The Cs and Mn metals bind with one cyano group of each TCNQ and the two superstructures are equally packed, in spite of Cs (ionic radius 1.81 Å) being larger than Mn (covalent radius 1.39 Å-1.69 Å) and forming a larger complex. Importantly, for Cs–TCNQ 4 , relatively large domains ( Fig. 1e ) are easily obtained after metal deposition, indicating a strong tendency of Cs–TCNQ 4 to form stable structures. In contrast to Mn–TCNQ 4 , the preparation of Cs–TCNQ 4 domains does not require additional post-deposition annealing. Gas-phase calculations of metal-TCNQ 4 complexes We performed DFT calculations to rationalize the structural differences of the two metal complexes and the emergence of the distinctive chiral ordering. Our analysis includes gas-phase calculations of individual metal–TCNQ 4 units (complexes), simulations of periodically repeated units in the absence of the surface, and calculations of metal–TCNQ 4 units on Ag(100). Relaxed structures and charge density isosurfaces of individual gas-phase units are shown in Fig. 2 . The isosurfaces show that Cs donates its valence electron to TCNQ 4 , and the resulting ionic bond allows free rotations of the molecules around the Cs + ion ( Fig. 2a ), whereas for Mn, a rigid, directional coordination bond with the ligand molecules is established ( Fig. 2b ). Both metals yield a stable complex with the four TCNQ molecules, with metal–TCNQ 4 binding energies of 7.1 eV and 4.5 eV for Mn and Cs, respectively. However, different metal–N–C bonding angles of ~140° and ~180° are obtained for Cs and Mn. Moreover, because of the Cs larger ionic radius and its different bonding with N-ligands, the individual Cs complex is 2.72 Å larger than the Mn one. The different steric flexibility and structural stiffness of the metal–TCNQ 4 units revealed by these results have important consequences for the packing of the complexes. 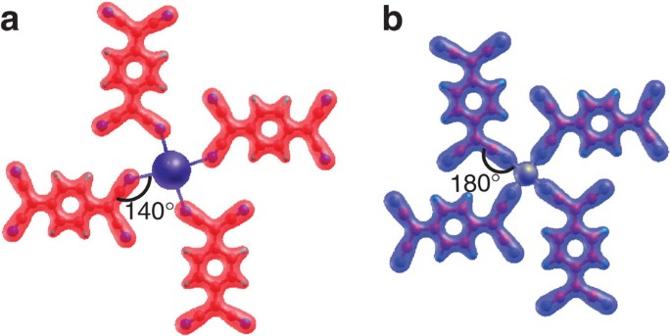Figure 2: Metal-TCNQ4electron density isosurface of isolated complexes calculated using DFT. (a) Cs–TCNQ4and (b) Mn–TCNQ4. In contrast to Mn that forms directional coordination bonds with TCNQ4, no charge is present around Cs. This shows that Cs fully donates its valence electron to the molecules establishing an ionic bond. The calculated diagonal distance between furthest N atoms is 25.18 Å and 22.46 Å for Cs–TCNQ4and Mn–TCNQ4,respectively. Figure 2: Metal-TCNQ 4 electron density isosurface of isolated complexes calculated using DFT. ( a ) Cs–TCNQ 4 and ( b ) Mn–TCNQ 4 . In contrast to Mn that forms directional coordination bonds with TCNQ 4 , no charge is present around Cs. This shows that Cs fully donates its valence electron to the molecules establishing an ionic bond. The calculated diagonal distance between furthest N atoms is 25.18 Å and 22.46 Å for Cs–TCNQ 4 and Mn–TCNQ 4, respectively. Full size image Gas-phase calculations of periodically repeated and relaxed chiral Cs–TCNQ 4 and achiral Mn–TCNQ 4 structures indicate that they are planar and stable at the experimental nearest-neighbour metal–metal distance ( Fig. 3 ) in comparison with structures calculated at other distances commensurate with the surface lattice vectors (6,1), (6,2), and (6,4). A comparison of the Mn–TCNQ 4 relaxed hypothetical chiral structure ( Fig. 3a , at the same experimental nearest-neighbour Mn–Mn distance) with the relaxed achiral superstructure ( Fig. 3b ) provides a first insight into the origin of the domain chirality observed experimentally. In the achiral structure, the outer, negatively charged TCNQ nitrogen atoms naturally avoid each other at an average distance of ~4.4 Å. This allows the complexes to remain planar after relaxation. However, in the chiral structure, the nitrogen atoms (highlighted by a red circle in Fig. 3a ) get too close to each other (~3.3 Å) if the units are constrained to a planar geometry. On full structural relaxation, their mutual repulsion is decreased by an out-of-plane buckling of the outer non-bonding cyano groups (of ~1 Å, Fig. 3a , down). Although the chiral and achiral configurations are energetically degenerate in gas-phase (within a few meV at the equilibrium inter-complex distance), the occurrence of buckling would be highly unlikely on the metal surface, as all cyano groups are expected to form a relatively strong bond with the underlying metal substrate [29] . Similar calculations performed for the chiral Cs–TCNQ 4 network reveal that the ~140° Cs–N–C bond angle allows an arrangement where the nitrogen atoms are sufficiently separated ( Fig. 3c ) to avoid each other without an out-of-plane buckling, hence resulting in a completely planar structure. 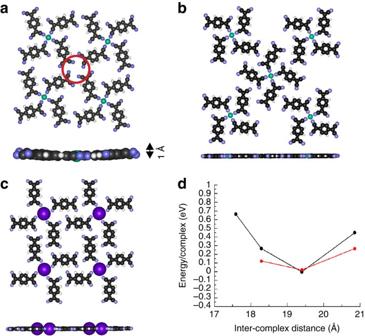Figure 3: Simulations of periodically repeated complexes in the absence of the surface. (a) Hypothetical chiral Mn–TCNQ4structure at the experimental distances of the achiral structure. The outer nitrogen atoms that repel each other and are buckled on relaxation are highlighted by a red circle. (b) Achiral Mn–TCNQ4structure observed in the experiment. The fully relaxed structure remains planar with the nitrogen atoms avoiding each other without causing an out-of-plane buckling. (c) Fully relaxed Cs–TCNQ4structure. In this case, the 140° Cs–N–C bonding angle allows the chiral configuration to remain planar. (d) Total energy per complex for free-standing Mn–TCNQ4chiral (black dots) and achiral (red dots) structures at commensurate surface distances, referred to the energy of the most stable structures. Figure 3: Simulations of periodically repeated complexes in the absence of the surface. ( a ) Hypothetical chiral Mn–TCNQ 4 structure at the experimental distances of the achiral structure. The outer nitrogen atoms that repel each other and are buckled on relaxation are highlighted by a red circle. ( b ) Achiral Mn–TCNQ 4 structure observed in the experiment. The fully relaxed structure remains planar with the nitrogen atoms avoiding each other without causing an out-of-plane buckling. ( c ) Fully relaxed Cs–TCNQ 4 structure. In this case, the 140° Cs–N–C bonding angle allows the chiral configuration to remain planar. ( d ) Total energy per complex for free-standing Mn–TCNQ 4 chiral (black dots) and achiral (red dots) structures at commensurate surface distances, referred to the energy of the most stable structures. Full size image A second effect favouring the formation of a Mn achiral structure is revealed by the comparison of the total energies between gas-phase achiral and hypothetical chiral structures at different inter-complex distances. Our calculations show that at non-equilibrium distances, the stress field developed by the chiral structure is substantially larger than in the achiral one ( Fig. 3d ). Given that STM measurements are performed at 300K, the relatively more flexible achiral structure will have a much higher (negative) entropy contribution to the free energy compared with the stiffer chiral packing due to vibrational entropy via thermally excited low-frequency phonons. Interaction of the complexes with the Ag(100) surface DFT calculations of Mn–TCNQ 4 ( Fig. 4a ) and Cs–TCNQ 4 ( Fig. 4b ) networks including the Ag(100) substrate strengthen all the arguments above in favour of the Mn–TCNQ 4 achirality and the Cs–TCNQ 4 network stability, and introduce new electrostatic ones. These calculations rule out the possibility of N-buckling: in both Cs and Mn complexes, we find that the outer nitrogen atoms form covalent bonds with the surface Ag atoms and reside at slightly different heights above the surface (~2.5 and 2.3 Å in the Mn and Cs networks ( Fig. 4c,d ), respectively). The model presented in Fig. 4a,c is the energetically most stable structure found among several configurations considered ( Supplementary Fig. S1 ). On structural relaxation, the pattern found in Fig. 4a and the analysis of the bonding charge (not shown) show that, for each TCNQ molecule, the two outer nitrogen atoms of the complex form bonds with Ag surface atoms. The nitrogen bound to the Mn centre, instead, exhibits significantly less pronounced bonding charge towards the substrate. The remaining nitrogen resides near a substrate hollow position, and does not contribute significantly to the adlayer–substrate bonding and to the corresponding energy decrease. One inter-complex hydrogen bond per TCNQ is formed in this structure. Comparing different geometries, we find that the binding energy is dominated by the number of N–Ag and of inter-complex hydrogen bonds present in the system (the intra-complex hydrogen bonds are the same in the different configurations considered). As found in the gas phase, the Mn atoms occupy the centre of their ligands' square arrangement, without deformation of the straight metal–ligand Mn–N–C bond alignment, which would be energetically too costly in this structure. Moreover, in the presence of the substrate, the experimentally observed achiral arrangement is 0.17eV/TCNQ more stable than the hypothetical chiral organization shown in Fig. 4e . This is easily rationalized: while in the former two N–Ag bonds/TCNQ and one inter-complex hydrogen bond per TCNQ are formed ( Fig. 4a ), in the latter, only one N–Ag bond/TCNQ is formed and no inter-complex hydrogen bond would be realized. In the homochiral structure, this is due to the Mn–N–C straight bonds leading to a repulsion of the negatively charged external nitrogen (having the same z coordinate above the substrate top-layer) that come close to each other. The reduction of this repulsion can only be achieved by a slightly rotated configuration, where only one N–Ag bond/TCNQ can be formed. The achiral arrangement can thus be simply rationalized as the only way to avoid the repulsive interaction between adjacent complexes without buckling the ligands and causing N–Ag bond breaking, to maximize the number of these bonds, and to favour the hydrogen-bond formation. In addition to these features, more pronounced finite temperature entropic effects further increase its stability relative to the chiral phase. 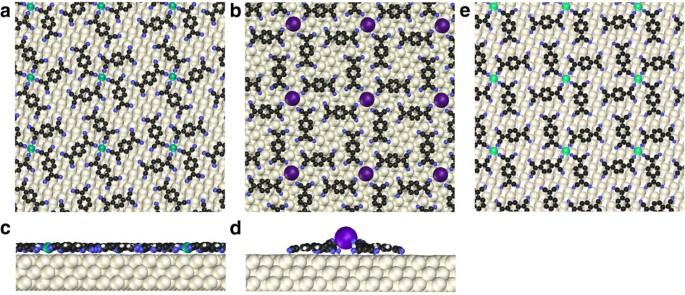Figure 4: Cs–TCNQ4and Mn–TCNQ4adlayers on Ag(100) surface. DFT models of the metal–TCNQ adlayers on Ag(100). (a,c) Planar Mn structure. (b,d) Highly non-planar, umbrella like Cs structure, with the Cs alkali atom substantially lifted up. (e) Hypothetical chiral Mn–TCNQ4structure. Figure 4: Cs–TCNQ 4 and Mn–TCNQ 4 adlayers on Ag(100) surface. DFT models of the metal–TCNQ adlayers on Ag(100). ( a , c ) Planar Mn structure. ( b , d ) Highly non-planar, umbrella like Cs structure, with the Cs alkali atom substantially lifted up. ( e ) Hypothetical chiral Mn–TCNQ 4 structure. Full size image The large, stable domains formed by the chiral Cs–TCNQ 4 units are ultimately made possible by the Cs–TCNQ bond flexibility, which yields relevant steric and electrostatic effects. Concerning the steric effects, the non-straight ~140° Cs–N–C bond angle, formed by virtue of the bond flexible character, allows the formation of two N–Ag bonds/TCNQ and, at the same time, of three inter-complex hydrogen bonds/TCNQ (a condition not realized in the Mn structure, which has only one such hydrogen bond). Moreover, the outer N atoms of the Cs–TCNQ 4 structure, being 0.2 Å closer to the Ag(100) surface than in the Mn-TCNQ 4 case, yield an expected increase of the N–Ag binding energy. We note that the ~140° Cs–N–C bond angle allows the Cs–TCNQ 4 units to be packed with the same assembly density of the Mn–TCNQ 4 domains, despite the individual unit being substantially larger. Metal–ligand charge transfer and surface dipole formation Further, significant differences in the relaxation pattern of the two metal–organic layers emerge from the calculations, indicating that the Cs-bonded TCNQ 4 adlayer is electrostatically more stable. We find that whereas the Mn–TCNQ 4 adlayer remains essentially flat on full structural relaxation (Mn and its ligand N atoms being at a height z =2.9 Å measured from the surface top layer, Fig. 4c ), the Cs–TCNQ 4 complexes become highly non-planar, with the Cs atoms significantly lifted up from the surface ( z =4.8 Å, Fig. 4d ) together with their bonding N atoms (average z =4.1 Å). This novel, out-of-plane 'umbrella'-like structure results in a laterally more compact, ordered arrangement, hosting a regular array of holes, as observed in the STM images in Fig. 1c,d . The structure has relevant effects on the surface electric dipole, which can be understood by considering the ionic nature of the Cs–TCNQ bond. To develop further insight on the relation between the different bonding patterns and the relative electrostatic stability of the Cs–TCNQ 4 and Mn–TCNQ 4 adlayers, we next analyse their electron density displacement field DF(x,y) , defined as , where: where z sub defines a plane dividing substrate and adlayer. This quantity represents the electron density of the interacting system ( ρ ) minus the densities of its three constituents (TCNQ molecules, bridging metal atoms and Ag substrate, in their electrically neutral state) calculated separately, but in the geometry they have in the interacting system. The field is illustrated in Fig. 5 . The coordination bonding electron density displacement pattern is clearly visible in the left panel at the bridging Mn sites, whereas the black depletion zones on the right panel reveal the complete ionization of the Cs atoms, which provides the molecular adlayer an additional rotational degree of freedom to achieve a stable assembly structure. 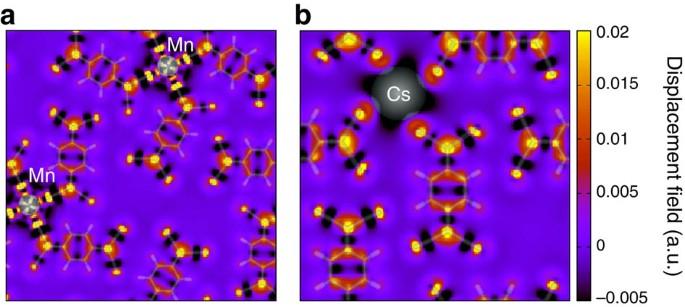Figure 5: Charge density displacement field. (a) Mn–TCNQ4and (b) Cs–TCNQ4. The plots account for the difference of electron charge density between the fully interacting system and its non-interacting components (see text). Positive charge (yellow, red) values indicate charge accumulation during the bonding process, highlighting, for example, the LUMO states of the TCNQ molecules (electronic acceptors). Negative values (black) refer to charge depletion. The structure model is superposed to the plots. Figure 5: Charge density displacement field. ( a ) Mn–TCNQ 4 and ( b ) Cs–TCNQ 4 . The plots account for the difference of electron charge density between the fully interacting system and its non-interacting components (see text). Positive charge (yellow, red) values indicate charge accumulation during the bonding process, highlighting, for example, the LUMO states of the TCNQ molecules (electronic acceptors). Negative values (black) refer to charge depletion. The structure model is superposed to the plots. Full size image We next note that charge transfer from the surface (CTS) to the adlayer is expected in this system. TCNQ has a large electronic affinity (that we calculate to be 3.49 eV), and the clean Ag(100) work function is 4.64 eV. The moderate 0.95 eV difference between these two values, possibly reduced by 'pillow effects', points to a likely charge transfer screened by polarization of the substrate and the TCNQ molecules themselves [8] ('image charge effect'). We also note that the Cs–TCNQ 4 stoichiometry of the assembly is too unbalanced for the Cs-donated electron to suffice for fully charging up each TCNQ anion, and to keep the neutrality of the 'organic salt' adlayer. Therefore, CTS is expected for the Cs- as well as for Mn-bridged TCNQ 4 adlayers, in both cases resulting in an overall negative surface electric dipole, whose value is ultimately limited by its own electrostatic cost. Interestingly, our DFT-calculated CTS for the Cs and Mn complexes is −0.39 e /TCNQ and −0.33 e /TCNQ, respectively. This indicates that the total charge acquired by each TCNQ in the Cs complex (estimated as −0.64 e /TCNQ, including the −0.25 e /TCNQ donated by Cs atoms) can be significantly larger than for Mn, suggesting that the Cs centres are better suited to the TCNQ electronegative character. Further calculations reveal a –2.67 D/TCNQ electric dipole for the Cs–TCNQ 4 adlayer, smaller in absolute value than the –2.75 D/TCNQ dipole associated with the Mn-bonded adlayer. Separate calculations carried out on the isolated neutral adlayers (in their adsorbed geometry, without including the metal surface) yield dipole values of +2.20 D/TCNQ and +1.44 D/TCNQ for the Cs and Mn structures, respectively. Thus, the dipole induced by the interaction with the surface is –4.77 D/TCNQ (–4.00 D/TCNQ) for the Cs (Mn) –adlayer. Clearly, a large cancellation occurs in the alkali metal-bonded adlayer between the positive dipole owing to the 'lifted up' Cs cations and the negative dipole induced by the CTS. A direct consequence is that a higher charge transfer on TCNQ and a smaller electric dipole can be achieved at the same time. All these results indicate that the highly non-planar assembly structure of the Cs–TCNQ 4 complexes, achievable by virtue of the flexible Cs–TCNQ bond and the relatively large Cs ionic radius implies an overall smaller negative-pointing surface dipole than in the Mn–TCNQ 4 case: a smaller surface dipole, in turn, stabilizes the Cs–TCNQ 4 supramolecular assembly owing to the lower electrostatic energy associated with the repulsion between individual complexes. More generally, our results suggest that alkali atom bridging can be useful to control the stability of self-assembled structures of electronegative organic molecules adsorbed on metal surfaces. For a start, a better steric performance of flexible units is induced by the ionic, rather than coordination, bonding. Furthermore, the stability is enhanced by electrostatic effects. Indeed, the TCNQ molecules will be allowed to become negatively charged well beyond the charge contribution provided by the alkali donor, and will thus repel each other as a layer of parallel adjacent negative dipoles. However, the electrostatic cost associated with the repulsion between Cs–TCNQ 4 units will be moderated by the strong positive local dipoles that develop at the alkali atom site within each unit, simply because of their increased height. The height increase will, in turn, favour further CTS. This interpretation suggests that the supramolecular adlayer stability and its overall state of charge could be further fine-tuned by different choices of alkali bridging ions. Combining experimental (STM) and theoretical (DFT) methods, we have shown that the chirality and relative stability of metal–organic supramolecular assemblies on a metal surface is strongly dependent on the choice of the bridging atom, yielding large chiral Cs–TCNQ 4 domains and achiral islands of Mn–TCNQ 4 complexes on a Ag(100) substrate. DFT calculations show that while the Mn–N coordination bonds are directional, rigid and poorly deformable, the Cs–N bonds are ionic, non-directional and highly flexible. The adlayer structure and global chirality are steered by intracomplex interactions and metal–ligand bonding: switching from directional coordination (Mn–TCNQ 4 ) to flexible ionic bonding (Cs–TCNQ 4 ) results in the switch from achiral to chiral domains. Thus, the control of the intracomplex stiffness offers a route to steer long-range organizational chirality, possibly providing a tool for the chiral design of organic crystals. Furthermore, the alkali-bridging atom allows charge transfer to the electronegative admolecules within the adlayer, which, unlike CTS, acts as a stabilizing electrostatic effect yielding a two-dimensional alkali organic salt. Interestingly, the atomic relaxation of alkali ions screens the build-up of the surface electric dipole, allowing for extra CTS. This implies that the bridging atoms that are used to control the assembly have also a role in the fine-tuning, via dipole formation, of the molecular charging and, thus, of the overall electronic level alignment of the metal–organic system. The results of this work, connecting molecular charging and assembly properties, are particularly significant for the study of level alignment effects in metal–organic interfaces, of great interest in organic electronics [30] . Sample preparation and data acquisition Experiments were carried out in a home-built ultrahigh vacuum chamber with a base pressure of 5×10 −10 mbar. The Ag(100) substrate was prepared by cycles of Ar + sputtering and annealing to 750 K that lead to the formation of flat terraces separated by monatomic steps. TCNQ molecules (purity 98%, Aldrich) were deposited from a quartz crucible heated to 400 K, with the substrate kept at 300 K. The coverage was kept below one monolayer. The molecular adlayers were subsequently exposed to a beam of metal atoms. Mn was evaporated using an electron-beam heated evaporator at a flux of ~0.2 monolayer per 5 min, while the sample was kept between T Ag =300 to 400 K to enhance the assembly process. Cs was deposited by means of resistive heating of a thoroughly degassed alkali metal dispenser (purchased from SAES) onto the substrate held at 300 K. The stoichiometry of metal TCNQ was kept below 0.25 to avoid the formation of fully reticulated networks [24] . After preparation, the sample was imaged by STM in situ at room temperature. Typical scanning parameters of 0.1–0.5 nA and ±0.8–1.2 V were used for imaging. Ab-initio calculations DFT calculations with periodic boundary conditions were performed with the planewave–pseudopotential package Quantum-ESPRESSO [31] , using ultrasoft pseudopotentials with a wavefunction (charge) energy cutoff of 408 eV (4080 eV) and a GGA–PBE exchange–correlation functional [32] . Calculations of achiral 2×Mn–TCNQ 4 on Ag(100) structure were performed with a wavefunction (charge) energy cutoff of 204 eV (2040 eV). Brillouin-zone sampling included the k= γ point only. The lowest energy model was obtained by fixing the unit cell size to 27.4 Å, a value chosen to be the closest to the experimental value (28.1 Å) and commensurate to the Ag(100) lattice parameter according to a (9, 3/−3, 9) superstructure. The molecular orientations (given by the angles formed by the molecular long axes with the [011] substrate direction) were initially set to the measured angles (+19°/−19°). For the half-sized unit cell of the hypothetical homochiral structure, we used two Bloch k -points for a consistent sampling of the (doubled) Brillouin zone and energy comparison with the heterochiral structures. The homochiral model for the Cs–TCNQ 4 structure was obtained by fixing the unit cell size to 19.4 Å, a value that is commensurate to the Ag(100) lattice parameter according to a (6, 3/−3, 6) superstructure, and exactly matches the experimental value. The molecular orientation was initially set to the measured angle (+19°). The Ag(100) surfaces were modelled with three layers, allowing a vacuum (adlayer–surface distance) of ~10 Å. Forces were relaxed up to 0.26 eV/ Å. In the presence of the surface, only forces acting on the top layer and the adlayer atoms were relaxed. See Supplementary Information section for a description of the different molecular adlayer geometries considered. How to cite this article: Abdurakhmanova, N. et al . Stereoselectivity and electrostatics in charge-transfer Mn- and Cs-TCNQ 4 networks on Ag(100). Nat. Commun. 3:940 doi: 10.1038/ncomms1942 (2012).